Dual-comb spectroscopy based on quantum-cascade-laser frequency combs Dual-comb spectroscopy performed in the mid-infrared—where molecules have their strongest rotovibrational absorption lines—offers the promise of high spectral resolution broadband spectroscopy with very short acquisition times (μs) and no moving parts. Recently, we demonstrated frequency comb operation of a quantum-cascade-laser. We now use that device in a compact, dual-comb spectrometer. The noise properties of the heterodyne beat are close to the shot noise limit. Broadband (15 cm −1 ) high-resolution (80 MHz) absorption spectroscopy of both a GaAs etalon and water vapour is demonstrated, showing the potential of quantum-cascade-laser frequency combs as the basis for a compact, all solid-state, broadband chemical sensor. Optical frequency combs were first introduced in the context of frequency metrology to bridge the gap between radio frequencies and optical frequencies [1] . Since then, several spectroscopy techniques using frequency combs have been demonstrated in various parts of the optical spectrum [2] . In the context of molecular spectroscopy, dual-comb spectroscopy [3] , [4] , [5] , [6] , [7] , [8] , [9] was proposed as an intriguing form of Fourier transform spectroscopy technique, showing a dramatic reduction in measurement times. The mid-infrared part of the optical spectrum is of paramount importance for molecular spectroscopy as the fundamental rotovibrational bands of most light molecules lie in this spectral range, with absorption strength orders of magnitude higher than in the visible or near-infrared [10] . Different approaches have been pursued to obtain mid-infrared frequency combs [11] , directly using transition metals incorporated into chalcogenide hosts [12] , [13] or Thulium-doped silica fibre lasers [14] , or indirectly using nonlinear conversion of near-infrared frequency combs [15] , [16] , [17] , [18] , [19] , [20] . However, these techniques tend to lead to relatively large set-up footprints, with the exception perhaps of microresonator-based combs that recently achieved operation in the mid-infrared [21] , [22] , [23] . Another possibility is a dual-comb-based technique combined with Raman spectroscopy that has recently been demonstrated [24] , [25] . Consequently, in order to widen the applications of frequency combs to the mid-infrared region of the spectrum, a semiconductor-based mid-infrared dual-comb spectrometer is of high interest for its simplicity and compactness. Quantum-cascade-lasers (QCLs) [26] have become the standard semiconductor laser source available in the mid-infrared range, achieving continuous-wave operation at room temperature [27] with watts of output power [28] . As QCLs are based on intersub-band transitions exhibiting an atomic-like joint density of states, heterogenous stacks [29] of active regions can be combined, achieving very large spectral coverage [30] when based on individual broadband active regions designs [31] . Fundamental mode-locking of QCLs has led to intense discussion in the literature [32] , [33] , [34] . Mode-locked operation of QCLs is difficult to achieve but have been demonstrated at cryogenic temperatures in the mid-infrared in a design where the upper-state lifetime was significantly increased using a highly diagonal laser transition [32] and in the terahertz where that lifetime is naturally much longer [35] . Recently, we have demonstrated room temperature, frequency comb operation of a QCL [36] with frequency-modulated (FM) output characteristics. In this work, we present a compact, semiconductor-based, electrically driven dual-comb spectrometer based on QCL frequency combs. As a proof of principle, we demonstrate broadband high-resolution absorption spectroscopy of a GaAs etalon showing broad absorption features as well as of water vapour at atmospheric pressure. Furthermore, we use the dual-comb set-up to demonstrate the equidistance of the comb teeth down to the mHz level. Mid-infrared QCL frequency combs Optical frequency combs are characterized by their perfectly equally spaced modes in the frequency domain, in which each individual comb line can be expressed as f n = f ceo + nf rep , where n is an integer, f rep is the comb line spacing (also called intermode beat) and f ceo is the carier-envelope offset frequency. As discussed in our previous work [36] , the phase-locking mechanism of a free-running, continuous-wave broadband QCL was identified to be four-wave mixing [37] , which, combined with the short gain recovery time of a QCL, leads to a phase signature comparable to a FM laser. This interpretation has been recently confirmed by simulations of the mode dynamics using Maxwell–Bloch equations [38] . Nevertheless, a flat broadband gain as well as a very low group velocity dispersion are required to achieve phase-locking. In this work, we employ two QCL frequency combs based on an InGaAs/InAlAs broadband design. They achieve continuous-wave operation at room temperature with several mWs of output power. The comb line spacing of a QCL comb is determined by the length of the device and by its group refractive index. Therefore, the comb line spacing can be easily fixed between few GHz (long devices) up to several tens of GHz (short devices). We used 6-mm-long devices, corresponding to comb line spacings of ~7.5 GHz (0.25 cm −1 ). The optical spectra of the combs are measured with a Fourier transform infrared spectrometer (0.12 cm −1 resolution) and are represented in Fig. 1a . The combs span 50 cm −1 with a comb line spacing of 0.25 cm −1 , resulting in 200 lines for each comb. In contrast to conventional frequency combs based on mode-locked lasers, the optical spectrum of FM combs does not show a gaussian envelope [7] , rather a complex amplitude distribution. 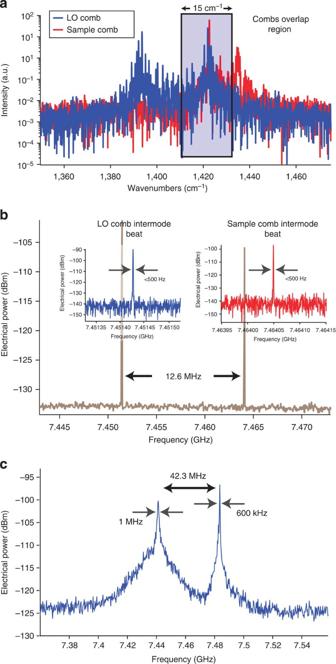Figure 1: QCL frequency combs beat notes. (a) Optical spectrum of the local oscillator (LO) comb (blue) and the sample comb (red) measured with a Fourier transform infrared spectrometer (FTIR; 0.12 cm−1resolution).ILO=544 mA,T=−13.25 °C andISignal=568 mA,T=4 °C. The combs overlap region of the spectrum spans over 15 cm−1. (b) Electrical intermode beat of the LO and signal combs in the so-called comb regime, measured with a spectrum analyser (span=30 MHz, RBW=3 kHz). Insets: same measurement with a higher resolution (span=200 kHz, RBW=500 Hz). (c) Electrical intermode beat of LO and signal combs in a high phase-noise regime, measured with a spectrum analyser (span=200 MHz, RBW=20 kHz). Figure 1: QCL frequency combs beat notes. ( a ) Optical spectrum of the local oscillator (LO) comb (blue) and the sample comb (red) measured with a Fourier transform infrared spectrometer (FTIR; 0.12 cm −1 resolution). I LO =544 mA, T =−13.25 °C and I Signal =568 mA, T =4 °C. The combs overlap region of the spectrum spans over 15 cm −1 . ( b ) Electrical intermode beat of the LO and signal combs in the so-called comb regime, measured with a spectrum analyser (span=30 MHz, RBW=3 kHz). Insets: same measurement with a higher resolution (span=200 kHz, RBW=500 Hz). ( c ) Electrical intermode beat of LO and signal combs in a high phase-noise regime, measured with a spectrum analyser (span=200 MHz, RBW=20 kHz). Full size image A very unique feature of QCL combs is the fact that the comb line spacing can be measured as an RF modulation arising directly on the laser-biasing current, and extracted from the device through a bias-tee. In fact, the electronic population dynamic in QCLs has an extremely high bandwidth because of the short intersub-band lifetimes (0.6 ps). Any RF modulation of the optical field is therefore reflected on the electronic population and thus on the current. We therefore found a clear correspondence between the comb line spacing measured electrically and with an optical detector [35] , [36] . The intermode beat notes of the two frequency combs measured with a spectrum analyser are shown in Fig. 1b . We observe a first intermode beat at 7.451 GHz and the second at 7.464 GHz, spaced by 12.6 MHz. Both intermode beats show extremely narrow linewidths (<500 Hz, resolution bandwidth (RBW) limited), which is a signature of the phase-locking mechanism of the combs. As a reference, we also drove the lasers in a high phase-noise regime by increasing the laser current [36] . This is the configuration encountered in conventional Fabry–Pérot devices [33] , [39] . The intermode beat is displayed in Fig. 1c and shows a high phase-noise pedestal (few MHz wide), with a lower phase-noise peak. The spacing between the two intermode beat note frequencies was increased in this regime in order to better separate them. 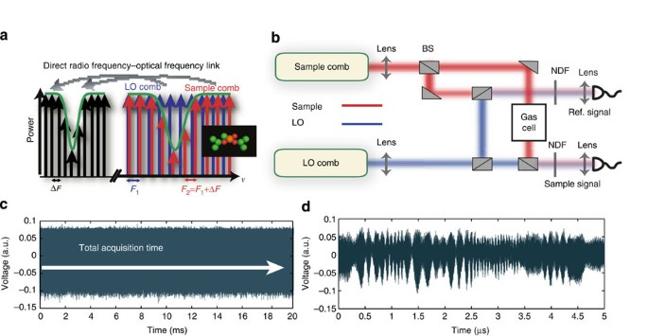Figure 2: Principle of dual-comb spectroscopy. (a) A multi-heterodyne beat of two frequency combs with slightly different comb spacings is created on a fast detector, generating a direct link between the optical and the RF domain. The multi-heterodyne beat signal contains information on the sample absorption. (b) Schematic view of the dual-comb spectroscopy set-up based on QCL frequency combs. One comb is used as a LO, while the other interrogates the gas cell. BS: 50–50 Antireflection-coated beam splitter, NDF: neutral density filter. (c) Typical time domain interferogram generated by a multi-heterodyne beat created by the beating of two QCL frequency combs. The beating of our two FM combs shows an almost constant amplitude. (d) Expanded version (4,000 times) of the same time domain interferogram. Multi-heterodyne beat and dual-comb spectroscopy Figure 2a shows a schematic of the principle of dual-comb spectroscopy. The technique is based on a multi-heterodyne beating of two frequency combs with slightly different comb line spacings ( f rep,1 and f rep,2 = f rep,1 +Δ f , respectively, where Δ f is the difference in the comb line spacings). A detector is then used to measure the multi-heterodyne beat. As shown schematically in Fig. 2a , each line of the first comb will beat with all lines of the second comb creating several different beats in the RF domain. Δ f must be chosen such as to obtain a one-to-one mapping between the lines of the two combs and their RF counterpart (see Supplementary Fig. 1 and Supplementary Note 1 ). Figure 2: Principle of dual-comb spectroscopy. ( a ) A multi-heterodyne beat of two frequency combs with slightly different comb spacings is created on a fast detector, generating a direct link between the optical and the RF domain. The multi-heterodyne beat signal contains information on the sample absorption. ( b ) Schematic view of the dual-comb spectroscopy set-up based on QCL frequency combs. One comb is used as a LO, while the other interrogates the gas cell. BS: 50–50 Antireflection-coated beam splitter, NDF: neutral density filter. ( c ) Typical time domain interferogram generated by a multi-heterodyne beat created by the beating of two QCL frequency combs. The beating of our two FM combs shows an almost constant amplitude. ( d ) Expanded version (4,000 times) of the same time domain interferogram. Full size image In most configurations of dual-comb spectroscopy [7] , one comb is used as a local oscillator, while the other is used to interrogate a sample, as shown in Fig. 2b . Owing to the one-to-one mapping, each multi-heterodyne beat contains information regarding the sample absorption at the optical frequency of the comb line interrogating the sample. As the technique relies on the discrete nature of a frequency comb, the sample absorption is measured at frequencies corresponding to the comb spacing (7.5 GHz=0.25 cm −1 ), defining thus the resolution. For the spectroscopy of large organic molecules or liquids, this resolution is usually sufficient. However, for gas spectroscopy of small molecules at low pressures, the molecule absorption lines are usually narrower (hundreds of MHz) than our comb spacing. As a special feature of QCL combs, the comb teeth can furthermore be swept over one comb spacing by tuning either its temperature or current. A dual-comb spectroscopy set-up is realized with the two QCL frequency combs previously described and is depicted in Fig. 2b (see Methods for further details). The difference in comb spacings Δ f can be set between 5 and 40 MHz by changing the temperature and current of both combs. The overlap region between the two combs spans around 15 cm −1 and is represented in Fig. 1a . We implemented a dual detection technique as it helps to remove technical noise on the detected amplitude [40] . No optical filter was used to spectrally select the overlap region. Note that the overlap region could be increased by using better-matched devices (using, for example, adjacent chips on the wafer, which was not the case for this work). The output power of the lasers is ~5 mW and the power on the detector is in general tens of μW as the beams are attenuated before the detection, to minimize detector nonlinearities. A typical time domain interferogram generated by a multi-heterodyne beat of the two QCL combs is shown in Fig. 2c,d . As opposed to the interferogram of conventional dual-comb set-ups where a burst at zero delay time is observed [7] , the beating of our two FM combs shows an almost constant amplitude. 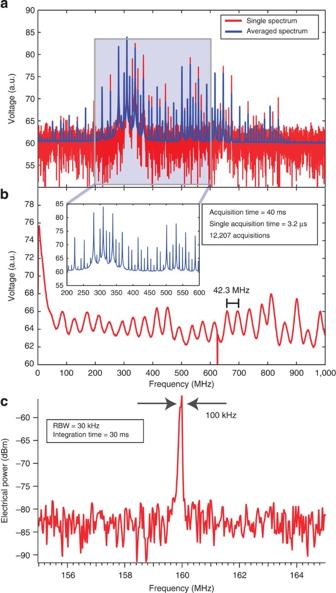Figure 3: Multi-heterodyne beat spectra. (a) Single multi-heterodyne spectrum (τacq=3.2 μs; red) and averaged (blue) multi-heterodyne spectrum (total acquisition time=100 ms, averaged over 30,517 samples) acquired with two QCLs in the comb regime (intermode beat spectrum shown inFig. 1b). (b) Averaged multi-heterodyne spectrum (total acquisition time=40 ms, averaged over 12,207 samples) where the two lasers are driven in an increased phase-noise regime (seeFig. 1c). Inset: zoom of the averaged multi-heterodyne spectra of two QCLs driven in the comb regime. (c) Single line of the multi-heterdoyne beat spectrum displayed inFig. 3a, measured with a spectrum analyser (sweep time=30 ms, RBW=30 kHz). Figure 3a shows a single multi-heterodyne spectrum (acquisition time τ acq =3.2 μs, in red) as well as an averaged multi-heterodyne spectrum (total acquisition time=100 ms, averaged over 30,517 spectra, in blue), where Δ f =9.58 MHz. A detailed description of data analysis used for computing the multi-heterodyne spectrum is given in the Supplementary Methods . The multi-heterodyne spectrum of the two combs spans 900 MHz with around N ~100 lines spaced by Δ f =9.58 MHz, corresponding to an optical bandwidth of ~25 cm −1 . Several beat notes can already be observed on the multi-heterodyne spectrum acquired over τ acq =3.2 μs. Figure 3: Multi-heterodyne beat spectra. ( a ) Single multi-heterodyne spectrum ( τ acq =3.2 μs; red) and averaged (blue) multi-heterodyne spectrum (total acquisition time=100 ms, averaged over 30,517 samples) acquired with two QCLs in the comb regime (intermode beat spectrum shown in Fig. 1b ). ( b ) Averaged multi-heterodyne spectrum (total acquisition time=40 ms, averaged over 12,207 samples) where the two lasers are driven in an increased phase-noise regime (see Fig. 1c ). Inset: zoom of the averaged multi-heterodyne spectra of two QCLs driven in the comb regime. ( c ) Single line of the multi-heterdoyne beat spectrum displayed in Fig. 3a , measured with a spectrum analyser (sweep time=30 ms, RBW=30 kHz). Full size image In order to achieve high signal-to-noise (SNR) ratio, the single acquisition time τ acq =3.2 μs should be shorter than the relative coherence time τ rel between the two combs, equal to inverse of the linewidth of an individual multi-heterodyne beat note. As shown in Fig. 3c , the latter is 100 kHz with a sweep time of 30 ms, corresponding to τ rel =10 μs. As this relative coherence time is expected to grow significantly with shorter acquisition time, our condition τ acq ≪ τ rel for coherent accumulation of the signal is well satisfied. Note also that the acquisition time τ acq =3.2 μs satisfies the condition τ acq >2/Δ f =158 ns needed to resolve the individual multi-heterodyne beat notes. We could therefore average all the multi-heterodyne spectra after aligning them numerically (see Supplementary Fig. 2 and Supplementary Methods ). As shown in Fig. 3a , all the individual beat notes are visible and above the noise floor on the averaged multi-heterodyne spectrum, demonstrating the high sensitivity of such a multi-heterodyne technique, with more than 50 dB in difference in power between the different beat notes. The heterodyne efficiency is difficult to be evaluated because of the important line-by-line amplitude variation. It is likely that the SNR ratio of this measurement can still be increased by improving the beam quality on the detector. To investigate the applicability of the results of ref. 41 to broadband spectroscopy, we measure the multi-heterodyne beat when both QCLs are driven in a high phase-noise regime. Figure 3b shows the multi-heterodyne spectrum in this configuration (here Δ f =42.3 MHz, as in Fig. 1c ). As a result of the additional phase-noise, the different multi-heterodyne beat notes display a large overlap, introducing an important cross talk between them. Increasing the frequency difference between the two comb spacings would address this issue at the cost of a much reduced optical frequency coverage. While narrowband spectroscopy has been successfully demonstrated with Fabry–Pérot devices operated in a high phase-noise regime [41] , our measurement demonstrates the advantage of QCL frequency combs for dual-comb spectroscopy rather than conventional Fabry–Pérot devices. Noise properties The multi-heterodyne set-up serves not only as a spectroscopic tool but also allows for the quantification of important comb characteristics using metrologically accepted counting techniques [21] . Since this set-up effectively maps down the frequency comb from optical domain to the RF frequencies, it allows to measure the equidistance of individual comb lines using frequency counters. The uniformity of the mode spacing can be quantified by evaluating the deviation from equidistant mode spacing ε, defined as [21] : Where f 0 , f N and f M are the frequencies of three multi-heterodyne beat notes. In our measurement, we have set Δ f =8 MHz, giving f 0 =30 MHz, N =5, f N =70 MHz, M =18 and f M =158 MHz. The set-up is illustrated in Fig. 4a (see Methods for further details). After detecting the multi-heterodyne beat signal, three electrical band-pass filters are used to isolate the beat notes at frequencies f 0 , f N and f M . After amplification, three frequency counters are used to measure the frequency oscillations of the beat notes. 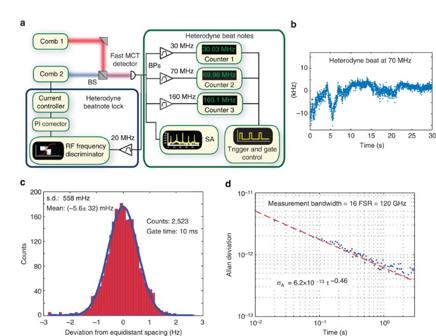Figure 4: Measurement of the deviation from equidistant mode spacing. (a) Schematic representation of the set-up used for measuring the deviation from equidistant mode spacing ε based on a multi-heterodyne measurement. SA, spectrum analyser; BPs, band-pass filters; BS, beam splitter; PI, proportional integral; MCT, mercury cadmium telluride. (b) Frequency oscillations of a single multi-heterodyne beat note when the slow drifts are corrected by the stabilization loop, measured with a frequency counter (total measurement time=30 s, gate time=10 ms). (c) Distribution of the deviation from equidistance mode spacingε. Total measurement time=25.23 s. Gate time=10 ms. The distribution shows a gaussian distribution with an average value of (−5.6±32) mHz and a s.d. of 558 mHz. (d) Allan deviation ofεnormalized by the total bandwidth of the measurement (16 × FSR=120 GHz). The Allan deviation shows an inverse square root dependency. Figure 4: Measurement of the deviation from equidistant mode spacing. ( a ) Schematic representation of the set-up used for measuring the deviation from equidistant mode spacing ε based on a multi-heterodyne measurement. SA, spectrum analyser; BPs, band-pass filters; BS, beam splitter; PI, proportional integral; MCT, mercury cadmium telluride. ( b ) Frequency oscillations of a single multi-heterodyne beat note when the slow drifts are corrected by the stabilization loop, measured with a frequency counter (total measurement time=30 s, gate time=10 ms). ( c ) Distribution of the deviation from equidistance mode spacing ε . Total measurement time=25.23 s. Gate time=10 ms. The distribution shows a gaussian distribution with an average value of (−5.6±32) mHz and a s.d. of 558 mHz. ( d ) Allan deviation of ε normalized by the total bandwidth of the measurement (16 × FSR=120 GHz). The Allan deviation shows an inverse square root dependency. Full size image In this experiment, we implement an active stabilization (by acting on the temperature of one device) to correct the slow frequency drifts of the multi-heterodyne beat spectrum, in effect to prevent them from drifting out of the bandwidth of the electrical filters (see Methods). Figure 4b shows the frequency oscillations of f N (centred at 70 MHz). The amplitude of the frequency drifts are less than 30 kHz over 30 s, which is significantly lower than the bandwidth of the filters. A precise control of both trigger and gate time of all the counters was implemented (see Methods). It is particularly important as any drift of f ceo will be seen as a nonuniformity of the comb line spacing if the counters are not perfectly synchronized. Even though the comb is not fully stabilized and f rep drifts, ε should be zero at any point of time for a perfectly synchronized set-up and a perfectly spaced comb. Figure 4c shows the distribution of ε over the entire measurement (gate time=10 ms, 2,523 counts). We measure a mean value of . Normalized to the optical carrier frequency (42.8 THz or 7 μm), this gives an accuracy of the equidistance of 7.5 × 10 −16 . The Allan deviation of ε is shown in Fig. 4d . These measurements definitely prove the equidistance of the mode spacing of a QCL frequency comb. Amplitude noise of each hererodyne beat note limits the sensitivity of a dual-comb absorption measurement. The SNR achieved with dual-comb spectroscopy has been investigated systematically in the context of conventional dual-comb spectroscopy by Newbury et al. [40] While the latter analysis is also valid for our set-up, note, however, that dual-comb spectroscopy with FM combs has a fundamental advantage in terms of SNR since, for a given average power, we reduce the peak power incident on the detector, improving therefore the available dynamical range. The amplitude noise of each of the multi-heterodyne beat notes from the spectra shown in Fig. 5a are investigated. 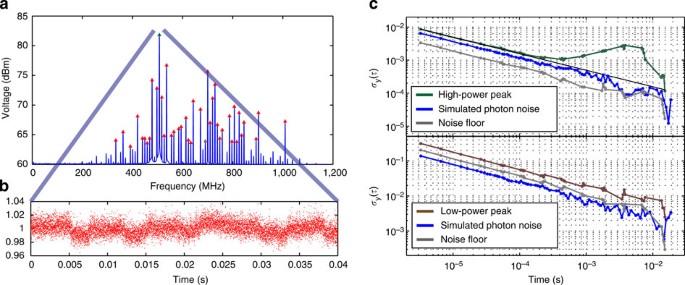Figure 5: Amplitude noise of the multi-heterodyne beat notes. (a) Multi-heterodyne spectra used for the amplitude noise measurement. The peak numbers 11 and 24 are highlighted as they were used for the amplitude noise characterization. (b) Amplitude oscillations of the amplitude of the highest amplitude beat note, normalized by its mean value (11th peak, in green). The time resolution of the measurement is again set to 3.2 μs. (c) Top: normalized Allan variation of the amplitude variations of the highest amplitude beat notes (11th peak, in green) as a function of the integration time. Bottom: normalized Allan variation of the amplitude variations of the low-amplitude beat notes (24th peak, in brown) as a function of the integration time. In both graphs we represent the Allan deviation of the amplitude variations induced by the detection noise floor and by the simulated photon noise. Figure 5b shows the normalized amplitude oscillations of the beat note having the highest amplitude as a function of time, corresponding to the 11 (green-marked) peak highlighted on Fig. 5a . We observe slow fluctuation on top of high frequency noise, with an amplitude of roughly 3%. The Allan deviation of the normalized amplitude oscillations of the highest and one of the lowest amplitude beat notes are shown in Fig. 5c as a function of the integration time (40 ms of total acquisition time). In addition, we represent the Allan deviation induced by the noise floor as well as by the photon noise (see Methods, Supplementary Fig. 3 and Supplementary Note 2 ). These measurements reveal that the magnitude of the amplitude noise of the multi-heterodyne beats is close to the shot noise limit, as shown on both plots on Fig. 5c . In both cases, we observe that the Allan deviations decrease with the integration time. However, the Allan deviation of the high amplitude peak increases at ~200 μs, corresponding to a technical noise that can be related to the low frequency oscillation observed in Fig. 5b . As the sensitivity of the low-amplitude peak is no longer sufficient to observe this technical noise, the corresponding Allan deviation decreases monotonically with the integration time. Although these measurements do not allow a direct evaluation of the importance of mode partition noise [42] , the fact that our experimental data lie close to simulations where only shot noise is taken into account indicates that mode partition noise adds, in the worst case, only 5–10 dB to the SNR of the system. These measurements prove that the QCL-based dual-comb set-up is an efficient spectroscopic tool with a SNR close to shot noise limit. Figure 5: Amplitude noise of the multi-heterodyne beat notes. ( a ) Multi-heterodyne spectra used for the amplitude noise measurement. The peak numbers 11 and 24 are highlighted as they were used for the amplitude noise characterization. ( b ) Amplitude oscillations of the amplitude of the highest amplitude beat note, normalized by its mean value (11th peak, in green). The time resolution of the measurement is again set to 3.2 μs. ( c ) Top: normalized Allan variation of the amplitude variations of the highest amplitude beat notes (11th peak, in green) as a function of the integration time. Bottom: normalized Allan variation of the amplitude variations of the low-amplitude beat notes (24th peak, in brown) as a function of the integration time. In both graphs we represent the Allan deviation of the amplitude variations induced by the detection noise floor and by the simulated photon noise. Full size image Broadband high-resolution spectroscopy As a first test of broadband spectroscopy, we first measure the transmission T of a low-finesse etalon consisting of a 450 μm-thick GaAs double-sided polished wafer. With a refractive index of ~3.3 at 7 μm wavelength, a 450 μm-thick GaAs etalon shows a periodic transmission with a period of 3.3 cm −1 . As discussed before, the etalon transmission acquired by our dual-comb set-up will be sampled at the comb spacing ~0.25 cm −1 . We therefore improved the resolution of our set-up by performing a frequency sweep of the combs and interleaving several spectra (see Supplementary Fig. 4 and Supplementary Methods ). Note that because we measure the frequency tuning of the LO and sample combs directly in the electrical domain, the frequency accuracy of the measurement is equal to the long-term stability of a single laser, that is, below 10 MHz. For practical reasons concerning this frequency sweep, the QCL combs had to be operated in a temperature region where the overlap spectra was 15 cm −1 rather than 25 cm −1 . 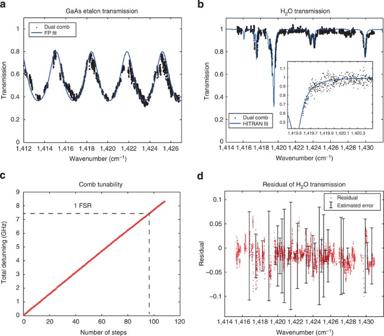Figure 6: Dual-comb transmission spectra. (a) GaAs Etalon transmission spectrum measured with our dual-comb spectrometer (0.25-cm−1comb spacing swept with a 80-MHz step) together with a fit based on the expression of the transmission of an etalon. (b) Water vapour transmission spectra in air (, total pressurePtot=101.3 kPa,T=20 °C) measured with our dual-comb spectrometer (800 MHz of spectral resolution after averaging) and HITRAN simulation. Inset: expansion of the measured transmission over ~1 cm−1with the full resolution (80 MHz). (c) Values of frequency tuning of the sample comb for each step of the tuning. The total detuning exceeded the bandwidth corresponding to the value of one comb line spacing (~7.5 GHz). (d) Residual between the water vapour transmission and the simulation using HITRAN database as well as the estimated errorσT. Figure 6a shows the transmission of the etalon measured with our dual-comb spectrometer (0.25 cm −1 comb spacing swept with a 80-MHz step), together with a fit performed using the expression of the transmission of an etalon. The fitting algorithm uses the etalon length L as fitting parameter and assumes fixed values for the refractive index of the material. We observe the periodic transmission of the etalon over a bandwidth of 15 cm −1 . The value of the etalon length computed by the fitting algorithm is 446 μm, in agreement with the measured thickness. The QCL combs are not actively stabilized while the transmission measurement is performed and slow drifts are still detrimental for the quality of the interleaved transmission. Figure 6: Dual-comb transmission spectra. ( a ) GaAs Etalon transmission spectrum measured with our dual-comb spectrometer (0.25-cm −1 comb spacing swept with a 80-MHz step) together with a fit based on the expression of the transmission of an etalon. ( b ) Water vapour transmission spectra in air ( , total pressure P tot =101.3 kPa, T =20 °C) measured with our dual-comb spectrometer (800 MHz of spectral resolution after averaging) and HITRAN simulation. Inset: expansion of the measured transmission over ~1 cm −1 with the full resolution (80 MHz). ( c ) Values of frequency tuning of the sample comb for each step of the tuning. The total detuning exceeded the bandwidth corresponding to the value of one comb line spacing (~7.5 GHz). ( d ) Residual between the water vapour transmission and the simulation using HITRAN database as well as the estimated error σ T . Full size image As a proof of principle applied to gas sensing, we performed transmission measurement of water vapour in air at atmospheric pressure in a 6-cm-long gas cell. We applied the same frequency sweep to the combs as described below (80 MHz step over a bandwidth equal to one comb line spacing). In order to avoid parasitic fringes coming from residual reflectivities in the beam path, we measured the multi-heterodyne beat signal with the gas cell filled with water vapour and subsequently with nitrogen, at each step of the frequency sweep. A reference measurement was thus taken at each step of the sweep and used to deduce the absolute value of the transmission. Figure 6b shows the transmission of water vapour in air (partial pressure of water vapour in air , total pressure P tot =101.3 kPa, T =20 °C) measured with the dual-comb set-up as well as a transmission simulation using HITRAN database [43] (see Methods). Figure 6c shows the frequency sweep applied to the sample comb, measured on the multi-heterodyne beat signal. The wavenumber scale calibration was carried out by using the HITRAN simulation and by applying a rigid shift to the measured transmission spectrum in order to fit the HITRAN simulation spectrum (see Supplementary Methods ). Over the entire duration of the measurement (few hours), the slow drifts reduce the quality of the interleaved transmission spectrum and a moving average filter was used for smoothing the interleaved transmission spectrum, reducing the effective resolution to 800 MHz. A typical interleaved spectrum contains ~5,000 points and the length of the filter was set to 11 points (see Supplementary Methods ). A clear agreement between the two measurements is observed over the entire measurement bandwidth (16 cm −1 ) and the absolute value of the transmission could also be retrieved. Owing to the important attenuation of the comb lines situated in the vicinity of the water absorption lines, their attenuated amplitude could lie below the noise floor of the detection set-up. In such a case, the algorithm calculating the absorption will not be able to retrieve the entire shape of the absorption line. This can be observed on the shape of the water absorption line situated at 1,419.5 cm −1 . Finally, as the multi-heterodyne spectrum presents beat notes with difference in amplitudes of more than 40 dB, the very low-intensity beat notes will not be detected by the algorithm calculating the absorption. This results in some holes on the spectrum and can also be observed on Fig. 6b , for instance, close to the water absorption line situated at 1,416.3 cm −1 . This issue could be resolved by sweeping the combs by more than one comb spacing. The residual between the water vapour measured with the dual-comb set-up and the HITRAN database simulation was also computed. Figure 6d shows the residual of all the points of the interleaved transmission spectrum together with the error estimated from the amplitude noise considerations (see Methods). The error calculation correctly predicts the residual between our measurement results and the HITRAN simulation, although the measurement is still clearly limited by technical noise. More importantly, the distribution of the residuals has a s.d. of 0.014, showing that our measurement has a precision of 1.4%. Compared with the transmission measurements demonstrated in ref. 41 , we have demonstrated that the comb operation of QCLs is crucial for achieving broadband multi-heterodyne spectroscopy. In conclusion, we have demonstrated a compact, semiconductor-based mid-infrared dual-comb spectrometer based on QCL frequency combs. We deeply characterized the noise properties of the dual-comb spectrometer. The experiment was also used to demonstrate the equidistance of the comb lines down to a fractional accuracy of 7.5 × 10 −16 . As a proof of principle, we have demonstrated broadband (16 cm −1 ) high-resolution (80 MHz=0.0027, cm −1 ) absorption spectroscopy of a low-finesse etalon as well as water vapour in air. These proof of principle experiments will encourage further development of instruments with much higher performances. Better-matched QCL combs implementing dispersion compensation [44] should enable a great increase in spectral coverage up to hundreds of cm −1 and decrease the peak-to-peak intensity variation. Better optics and detectors with a larger dynamical range will better deal with the line-to-line amplitude variation. Actively stabilization of both the frequency comb offset frequency and repetition frequency will also improve the SNR of our measurements as well as simplifying the data treatment. All-electrical measurements and stabilization of the repetition frequency of the laser could be carried out as the intermode beat note can be measured electrically. Our system holds the potential to achieve a monolithically integrated mid-infrared dual-comb spectrometer achieving ultrahigh sensitivity combined with broadband spectral coverage and high resolution, with applications in many fields such as personalized medicine, environment and process control. Dual-comb set-up The QCLs used to realize the dual-comb spectroscopy set-up were not cleaved together and therefore present different comb spacings. The difference between two comb spacings being , where n g is the group index, a difference of the two comb spacings Δ f ≤50 MHz corresponds, for a L =6-mm-long device, to a maximum length difference Δ L between the two devices of less than 40 μm. The frequency difference Δ f could be set between 5 and 40 MHz by controlling the current and/or temperature of each comb. Each comb is first collimated by an 1-inch f/1 aspheric lens. The sample to be investigated by our dual-comb spectroscopy set-up is injected in a gas cell (6-cm long with AR-coated 2-inch ZnSe windows). The gas cell is also placed in a motorized stage and can be moved out of the optical path. Otherwise, a low-finesse GaAs etalon is placed on the motorized stage. Both combs are heterodyned into a fast (590 MHz, 3 dB cutoff frequency) thermoelectric cooled (TEC) mercury cadmium telluride (MCT) photovoltaic detector (Vigo PV-4TE-10.6) giving the sample signal. For reference measurements (without sample), the sample and LO combs are both separated by 50–50 wedged beam splitters and heterodyned in a second identical detector without the influence of the investigated sample. The beams were attenuated by neutral density filters to avoid saturation of the detectors. Both signals are then acquired either with a spectrum analyser or by a 12-bit vertical resolution, 1 GHz analogue bandwidth, 2.5 GSample/s sampling frequency oscilloscope (memory of 250 MSamples for the XL memory option (used for Fig. 3a ) or 100 MSamples per channel for L memory option (used for all other figures)). Both sample signal and reference signal can be acquired with the same trigger on the two different channels of the oscilloscope. The entire set-up is placed in a nitrogen-purged environment. All technical sources of noise on the set-up were carefully investigated and reduced. Acoustic noise as well as temperature fluctuations of the room are reduced by placing the entire set-up into a box. Both lasers are driven with low noise current drivers (Wavelength electronics QCL1000) with a specified average current noise density of . In addition, a home-made battery system capable of driving both lasers for several hours was used. The temperature fluctuations of the lasers were also reduced to less than 10 mK by using a low thermal drift temperature controller (wavelength electronics PTC10K-CH) with a 50-kΩ thermistor. Measurement of the deviation from equidistance mode spacing The multi-heterodyne signal is detected by a fast MCT photovoltaic detector (Vigo PV-4TE-10.6). Three narrow bandwidth (5 MHz) band-pass filters centred at 30, 70 and 160 MHz are used to isolate the beat notes. Three frequency counters (Agilent 53220A) are used to count for the frequency oscillations of the beat notes. An active stabilization was implemented to perform a weak locking (~1 kHz bandwidth) for correcting the multi-heterodyne beat spectrum against the slow drifts. A band-pass filter (20 MHz centre frequency, 5 MHz bandwidth) was used to isolate a fourth beat note to be used as error signal. The frequency oscillations of this beat note were converted into amplitude oscillations through a RF frequency discriminator (Miteq FMDM-21.4/4-2B-R, centre frequency 21.4 MHz, 8 MHz bandwidth, 1 V MHz −1 sensitivity). The output of this RF frequency discriminator was used as the input of a Proportional Integral corrector (Zurich Instrument HH2LI-PID, 5 kHz bandwidth) acting on the current of one of the combs. High SNR (30 dB or more) beat notes were used for this experiment in order to be correctly detected by the frequency counters. The gate and the time control were controlled by a trigger (Agilent 33220 A, pulse mode). To verify that the counters were correctly synchronized, a FM signal with a slowly varying carrier frequency (carrier frequency 10 MHz, frequency deviation ~1 kHz, FM frequency ~1 Hz) was generated by a frequency generator (Agilent 33220 A, FM modulation mode) and counted by the three counters. The deviation from the equidistant spacing was measured and showed values at least one order of magnitude lower than the deviation from the equidistant spacing measured with the QCL combs. All the instruments where connected to the same 10-MHz clock reference. Allan deviation measurements The Allan deviation of the noise floor is evaluated by blocking the two beams, measuring the amplitude oscillations at the frequency of the corresponding beat note and normalizing these oscillations by the mean amplitude of the corresponding beat note. The Allan deviation of the photon noise accounts for the amplitude oscillations of the beat note in the case where the only noise source is the shot noise of the lasers (see Supplementary Note 2 ). HITRAN simulation The HITRAN 2008 database was used for the simulation of the transmission of water vapour in air. The partial pressure of water vapour in air used in the simulations is , the total pressure is P tot =101.3 kPa and the temperature is T =20 °C. The frequency resolution was set to 0.001 cm −1 . A Voigt profile was assumed and no instrumental lineshape was taken into account. Residual and error estimation The transmission of water vapour is related to the voltage generated by a heterodyne beat on the detector by: where T is the transmission, (respectively ) is the voltage generated by a multi-heterodyne beat with the gas cell filled with water vapour ( N 2 ). Therefore, any voltage oscillation of ( ), characterized by its s.d. ( ) influences the transmission t by: where σ t is the s.d. of the transmission. We assume that and we estimate by measuring the s.d. and the mean value of the voltage oscillations created by every heterodyne beat note, as shown in Fig. 5b . How to cite this article: Villares, G. et al. Dual-comb spectroscopy based on quantum-cascade-laser frequency combs. Nat. Commun. 5:5192 doi: 10.1038/ncomms6192 (2014).